ORMDL3 promotes eosinophil trafficking and activation via regulation of integrins and CD48 ORM (yeast)-like protein isoform 3 ( ORMDL3 ) has recently been identified as a candidate gene for susceptibility to asthma; however, the mechanisms by which it contributes to asthma pathogenesis are not well understood. Here we demonstrate a functional role for ORMDL3 in eosinophils in the context of allergic inflammation. Eosinophils recruited to the airways of allergen-challenged mice express ORMDL3. ORMDL3 expression in bone marrow eosinophils is localized in the endoplasmic reticulum and is induced by interleukin-3 and eotaxin-1. Overexpression of ORMDL3 in eosinophils causes increased rolling, distinct cytoskeletal rearrangement, extracellular signal-regulated kinase (1/2) phosphorylation and nuclear translocation of nuclear factor kappa B. Knockdown of ORMDL3 significantly inhibits activation-induced cell shape changes, adhesion and recruitment to sites of inflammation in vivo, combined with reduced expression of CD49d and CD18. In addition, ORMDL3 regulates interleukin-3-induced expression of CD48 and CD48-mediated eosinophil degranulation. These studies show that ORMDL3 regulates eosinophil trafficking, recruitment and degranulation, further elucidating a role for this molecule in allergic asthma and potentially other eosinophilic disorders. Several genome-wide association studies provide strong evidence that polymorphisms in the region including ORM (yeast)-like protein isoform 3 ( ORMDL3 ) on chromosome 17q21 contribute to childhood as well as adult-onset asthma in ethnically diverse populations [1] , [2] , [3] , [4] , [5] , [6] , [7] , [8] . The human ORMDL genes, which include ORMDL1 on chromosome 2, ORMDL2 on chromosome 12 and ORMDL3 on chromosome 17, are expressed ubiquitously in adult and fetal tissues, including the lung, with human ORMDL3 gene demonstrating 96% homology with mouse ORMDL3 (ref. 9 ). ORMDL3 gene encodes an endoplasmic reticulum (ER) trans-membrane protein that binds to sarco-ER Ca 2+ pump regulating ER-mediated Ca 2+ signalling and cellular stress by facilitating the unfolded-protein response in transfected HEK293 cells [10] . In addition, ORMDL3 functions as a mediator of sphingolipid homeostasis in yeast and changes in gene expression or mutations in its phosphorylation sites cause dysregulation of Ca 2+ homeostasis and sphingolipid metabolism [11] . Although genetic studies have clearly demonstrated that the ORMDL3 locus is a risk factor for asthma, the function(s) of ORMDL3 in mediating allergic airway inflammation is only now beginning to emerge. A recent study showed that ORMDL3 is an inducible, ER-expressed protein in bronchial epithelial cells where it regulates expression of metalloproteases and chemokines and that ORMDL3 may be linked to asthma via an ER unfolded-protein response pathway [12] . This study also demonstrated that mRNA for ORMDL3 is expressed by mouse bone marrow (BM)-derived eosinophils at significantly higher levels compared with ORMDL1 and ORMDL2 mRNA and that ORMDL3 protein is induced in bronchoalveolar lavage fluid (BALF) eosinophils of mice after allergen challenge. However, the function of this protein at a cellular level in leukocytes is not known. Interestingly, a recent case–controlled study in Korean children indicated a link between ORMDL3 gene variants and eosinophilic inflammation [13] . Eosinophils are the predominant inflammatory leukocytes that infiltrate airways and promote inflammation during allergic asthma [14] . Herein, we asked whether ORMDL3 has a role in regulating eosinophil trafficking, migration and recruitment as well as activation-dependent degranulation, which are critical events that support the development and maintenance of tissue inflammation during allergic asthma and other eosinophil-driven disorders. Our studies show that ORMDL3 has a role in promoting eosinophil trafficking and activation via regulation of integrins (CD49d and CD18) and CD48. Allergen challenge induces expression of ORMDL3 in the lungs Given the identification of ORMDL3 as a candidate gene associated with asthma, we first examined whether ORMDL3 expression was evident in murine lungs exposed to various allergens by immunohistology with a polyclonal antibody against human ORMDL3 that is known to react with mouse ORMDL3. Ability of this antibody to bind ORMDL3 was established by western blot analysis of bacterial lysates expressing recombinant human ORMDL3 (His-tagged) or recombinant mouse ORMDL3 (GST-tagged), which showed bands of ~17 kDa for His-ORMDL3 and ~43 kDa for GST-ORMDL3 fusion protein, respectively ( Supplementary Fig. S1a ), corresponding to the molecular weight of ORMDL3 (ref. 12 ). In lung sections, relative to control mice, where ORMDL3 expression was noted mostly in airway epithelial cells and endothelial cells by immunohistology ( Fig. 1a , middle panel), mice challenged with an extract of Alternaria alternata demonstrated ORMDL3 expression associated not only with airway epithelial cells and endothelial cells but also with inflammatory cells recruited to the allergic airways ( Fig. 1a , right panel). Western blot analysis of lung tissue lysates with this antibody further indicated increased expression of ORMDL3 in the lungs after exposure to Alternaria extract ( Supplementary Fig. S1b ). Exposure to other allergens such as ovalbumin (chronic exposure) or cockroach antigen (acute exposure) also showed ORMDL3 expression in leukocytes in the lungs of mice, although the level of expression is variable and likely to be allergen-specific ( Supplementary Fig. S2a ). As eosinophils are the major inflammatory cells recruited to the airways in response to Alternaria challenge ( Supplementary Fig. S2b ), we next examined whether eosinophils in the lung tissue of Alternaria -exposed mice express ORMDL3 by staining sequential lung sections for expression of ORMDL3 and eosinophil-specific major basic protein (MBP) with antibodies against ORMDL3 and MBP, respectively ( Fig. 1b ). Areas with several MBP-positive cells also stained positive for ORMDL3. In addition, dual immunofluorescence staining of BALF cells from Alternaria -exposed mice with these antibodies confirmed that MBP-positive cells (eosinophils) recruited to the airways express ORMDL3 ( Fig. 1c ). Expression of ORMDL3 by eosinophils was further validated in BM-derived murine eosinophils by RT–PCR (see Supplementary Table S1 for primer details) and western blot analysis, which demonstrated a major protein band of molecular weight ~17 kDa ( Fig. 1d ). Consistent with the pattern indicated for this antibody by the manufacturer, additional protein bands in the molecular weight range of ~45–70 kDa were noted. Owing to the significant homology between ORMDL proteins 1, 2 and 3 (>80%) [9] , one cannot unequivocally rule out that the antibody does not react with ORMDL1 or 2. However, previous studies indicating that ORMDL3 mRNA expression is induced in the lungs of mice challenged with interleukin (IL)-4 or IL-13 (Th2 cytokines expressed in response allergen challenge) and that BM-derived eosinophils express predominantly ORMDL3 mRNA relative to ORMDL1 and 2 (ref. 12 ) support our demonstration of ORMDL3 protein expression in Alternaria -challenged murine lungs and eosinophils with this antibody. 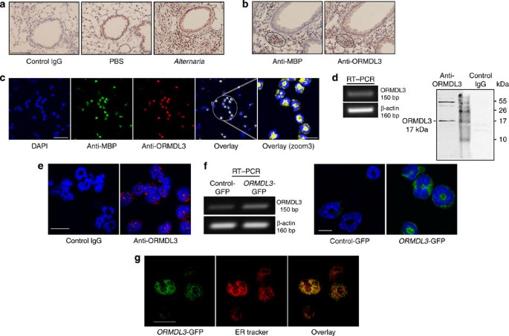Figure 1:ORMDL3 expression in lungs of allergen-challenged mice and BM-derived murine eosinophils. (a) Expression of ORMDL3 by airway epithelial cells, endothelial cells and recruited inflammatory cells in the lungs of mice challenged with an extract ofA. alternataby immunohistochemistry (IHC) with antibodies against ORMDL3 (right). Baseline ORMDL3 expression in lungs of PBS-exposed control mice (centre) and reactivity with control IgG (left) are also shown. Scale bar, 10 μm. (b) Peribronchial area in sequential lung sections exhibiting similar pattern of eosinophil-specific MBP (left) and ORMDL3 (right) expression by IHC (highlighted by the circle as an example). Scale bar, 10 μm. (c) Expression of ORMDL3 by eosinophils in BALF ofAlternaria-challenged mice by dual immunofluorescence staining with antibodies against MBP (green) and ORMDL3 (red) followed by confocal microscopy after labelling with DAPI (blue). Scale bar, 50 μm. A zoom three magnified image of cells highlighted by the circle in the overlay is shown (far right panel). Scale bar, 20 μm. (d) Expression of ORMDL3 in BM-derived murine eosinophils by RT–PCR with β-actin as the internal control (left panel) and by western blot analysis with antibodies against ORMDL3 (right panel, left lane). Molecular weight markers (centre lane) and binding of control IgG (right lane) are also shown. (e) Expression of ORMDL3 in DAPI-labelled BM-derived eosinophils by immunofluorescence staining with antibodies against ORMDL3 (right) or control IgG (left). Scale bar, 20 μm. (f) Expression of ORMDL3 in BM-derived eosinophils transfected withORMDL3-GFP or control-GFP by RT–PCR (left) and confocal microscopy (right). Expression of β-actin is shown as the internal control for the RT–PCR. Scale bar, 10 μm. (g) Sub-cellular localization of ORMDL3. Murine eosinophils were transfected withORMDL3-GFP (left) and then treated with ER-Tracker Red for live-cell ER labelling (middle). Co-localized expression ofORMDL3-GFP and ER-Tracker Red is shown in the overlay (right). Scale bar, 10 μm. Data are representative ofn=4 mice per group in (a–c) and of two to five independent experiments with BM-derived eosinophils from different mice in (d–g). Figure 1: ORMDL3 expression in lungs of allergen-challenged mice and BM-derived murine eosinophils . ( a ) Expression of ORMDL3 by airway epithelial cells, endothelial cells and recruited inflammatory cells in the lungs of mice challenged with an extract of A. alternata by immunohistochemistry (IHC) with antibodies against ORMDL3 (right). Baseline ORMDL3 expression in lungs of PBS-exposed control mice (centre) and reactivity with control IgG (left) are also shown. Scale bar, 10 μm. ( b ) Peribronchial area in sequential lung sections exhibiting similar pattern of eosinophil-specific MBP (left) and ORMDL3 (right) expression by IHC (highlighted by the circle as an example). Scale bar, 10 μm. ( c ) Expression of ORMDL3 by eosinophils in BALF of Alternaria -challenged mice by dual immunofluorescence staining with antibodies against MBP (green) and ORMDL3 (red) followed by confocal microscopy after labelling with DAPI (blue). Scale bar, 50 μm. A zoom three magnified image of cells highlighted by the circle in the overlay is shown (far right panel). Scale bar, 20 μm. ( d ) Expression of ORMDL3 in BM-derived murine eosinophils by RT–PCR with β-actin as the internal control (left panel) and by western blot analysis with antibodies against ORMDL3 (right panel, left lane). Molecular weight markers (centre lane) and binding of control IgG (right lane) are also shown. ( e ) Expression of ORMDL3 in DAPI-labelled BM-derived eosinophils by immunofluorescence staining with antibodies against ORMDL3 (right) or control IgG (left). Scale bar, 20 μm. ( f ) Expression of ORMDL3 in BM-derived eosinophils transfected with ORMDL3 -GFP or control-GFP by RT–PCR (left) and confocal microscopy (right). Expression of β-actin is shown as the internal control for the RT–PCR. Scale bar, 10 μm. ( g ) Sub-cellular localization of ORMDL3. Murine eosinophils were transfected with ORMDL3 -GFP (left) and then treated with ER-Tracker Red for live-cell ER labelling (middle). Co-localized expression of ORMDL3 -GFP and ER-Tracker Red is shown in the overlay (right). Scale bar, 10 μm. Data are representative of n =4 mice per group in ( a – c ) and of two to five independent experiments with BM-derived eosinophils from different mice in ( d – g ). Full size image Previous studies indicate that ORMDL3 is an ER membrane protein in transfected HEK293 (ref. 9 , 10 ) and A549 epithelial cells [12] . We examined sub-cellular localization of ORMDL3 in murine eosinophils by immunofluorescence staining. Expression was restricted largely to the cytoplasm ( Fig. 1e ). To further elucidate this, eosinophils were transfected with ORMDL3 -GFP (green fluorescent protein). RT–PCR with specific primers demonstrated increased ORMDL3 expression and confocal microscopy showed a fluorescent (GFP) signal localized to the cytoplasm in transfected eosinophils ( Fig. 1f ). ORMDL3 -GFP-transfected eosinophils ( Fig. 1g , left panel) stained with ER-Tracker Red ( Fig. 1g , middle panel) showed that GFP-tagged ORMDL3 expression overlapped with ER-Tracker Red staining ( Fig. 1g , right panel) indicating that ORMDL3 expression in eosinophils is predominantly confined to the ER, consistent with previous findings in epithelial cells. ORMDL3 is induced by IL-3 and participates in cell activation As exposure to allergens induces ORMDL3 expression in the lungs of mice, we evaluated whether expression of ORMDL3 at a cellular level in murine eosinophils is regulated by IL-3, IL-5, eotaxin-1 and RANTES that promote allergic asthma [14] . RT–PCR and qPCR indicated that IL-3 and eotaxin-1 markedly induce ORMDL3 expression, whereas IL-5 and RANTES had no effect ( Fig. 2a , top and bottom panel). Western blot analysis of eosinophil lysates demonstrated increased ORMDL3 protein expression after exposure to IL-3 ( Fig. 2b ), confirming its ability to upregulate ORMDL3 expression. In human eosinophils, IL-3 has been shown to induce rapid activation of extracellular signal-regulated kinase (ERK; 1/2) but not p38 (ref. 15 ). Likewise, eotaxin-1 has been shown to induce rapid activation of ERK (1/2) (p44/42) and p38 MAP kinases, which have a role in regulating eosinophil migration and degranulation [16] , [17] . As IL-3 and eotaxin-1 induced ORMDL3 expression, we examined whether overexpression of ORMDL3 is associated with activation of ERK and p38 in eosinophils. ORMDL3 -GFP-transfected eosinophils demonstrated a marked increase in levels of phosphorylated ERK (1/2) compared with non-transfected or control-GFP-transfected cells, whereas no effect was noted on the level of activated p38 ( Fig. 2c ). Activated ERK can induce nuclear translocation of NF-κB via activation of its cytoplasmic target I-κB kinase alpha (IKK-alpha) [18] . Therefore, we next examined if ORMDL3, when overexpressed, can regulate NF-κB expression and translocation in murine eosinophils. Overexpression of ORMDL3 in ORMDL3 -GFP-tranfected eosinophils (akin to IL-3- or eotaxin-1-induced ORMDL3 expression) resulted in translocation of NF-κB to the nucleus ( Fig. 2d ). Nuclear translocation and activation of NF-κB in eosinophils is known to induce expression of multiple proteins (such as cytokines and adhesion molecules) resulting in further cell activation [19] , [20] . 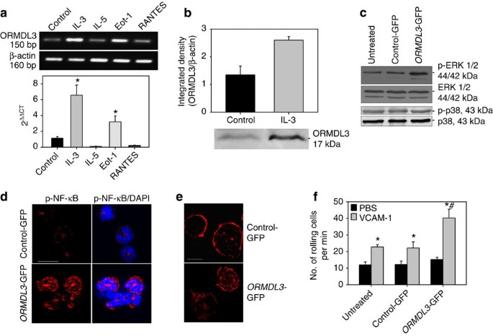Figure 2:IL-3- and eotaxin-1-induced expression of ORMDL3 by eosinophils and cell activation. (a) ORMDL3 expression in BM-derived eosinophils cultured in medium alone (control) or medium containing IL-5, IL-3, RANTES-1 (100 ng ml−1) or eotaxin-1 (Eot-1, 100 nM) for 2 h by RT–PCR (top) and qPCR (bottom). (b) ORMDL3 expression in eosinophils treated with IL-3 for 12 h by western blot analysis followed by densitometry. Densitometry data are normalized against expression of β-actin used as the internal control. ORMDL3 expression in representative control and IL-3-treated eosinophil lysates is shown below bar graph. (c) Levels of ERK (1/2), phospho-ERK (1/2), p38 and phospho-p38 in eosinophils transfected with control-GFP,ORMDL3-GFP or left untreated by western blot analysis. (d) NF-κB expression in DAPI-labelled control-GFP- andORMDL3-GFP-transfected eosinophils by immunofluorescence staining with antibodies against phospho-NF-κB p65. Scale bar, 10 μm. (e) Cytoskeletal arrangement in eosinophils transfected with control-GFP orORMDL3-GFP by confocal microscopy after phalloidin staining. Scale bar, 10 μm. (f) Rolling of murine eosinophils transfected with control-GFP orORMDL3-GFP on rm VCAM-1-coated cover-slips under conditions of flowin vitro. Data shown in (a,top) and (c–e) is representative of two to three independent experiments with eosinophils from different mice. Combined data (mean±s.e.m.) from three experiments in triplicate in (a,bottom) and two experiments in duplicate in (f) is shown. In (b), combined data (mean±s.d.) from two out of three experiments with similar results is shown. *P<0.01 in (a,bottom) compared with control and <0.02 in (f) compared with rolling on PBS;#P<0.05 in (f) compared with control-GFP. Statistical significance was determined by unpaired two-tailed Student’st-test. Figure 2: IL-3- and eotaxin-1-induced expression of ORMDL3 by eosinophils and cell activation . ( a ) ORMDL3 expression in BM-derived eosinophils cultured in medium alone (control) or medium containing IL-5, IL-3, RANTES-1 (100 ng ml −1 ) or eotaxin-1 (Eot-1, 100 nM) for 2 h by RT–PCR (top) and qPCR (bottom). ( b ) ORMDL3 expression in eosinophils treated with IL-3 for 12 h by western blot analysis followed by densitometry. Densitometry data are normalized against expression of β-actin used as the internal control. ORMDL3 expression in representative control and IL-3-treated eosinophil lysates is shown below bar graph. ( c ) Levels of ERK (1/2), phospho-ERK (1/2), p38 and phospho-p38 in eosinophils transfected with control-GFP, ORMDL3 -GFP or left untreated by western blot analysis. ( d ) NF-κB expression in DAPI-labelled control-GFP- and ORMDL3 -GFP-transfected eosinophils by immunofluorescence staining with antibodies against phospho-NF-κB p65. Scale bar, 10 μm. ( e ) Cytoskeletal arrangement in eosinophils transfected with control-GFP or ORMDL3 -GFP by confocal microscopy after phalloidin staining. Scale bar, 10 μm. ( f ) Rolling of murine eosinophils transfected with control-GFP or ORMDL3 -GFP on rm VCAM-1-coated cover-slips under conditions of flow in vitro . Data shown in ( a , top ) and ( c – e ) is representative of two to three independent experiments with eosinophils from different mice. Combined data (mean±s.e.m.) from three experiments in triplicate in ( a , bottom ) and two experiments in duplicate in ( f ) is shown. In ( b ), combined data (mean±s.d.) from two out of three experiments with similar results is shown. * P <0.01 in ( a , bottom ) compared with control and <0.02 in ( f ) compared with rolling on PBS; # P <0.05 in ( f ) compared with control-GFP. Statistical significance was determined by unpaired two-tailed Student’s t -test. Full size image Exposure of eosinophils to eotaxin-1 induces cytoskeletal rearrangement, which enables cells to undergo morphological changes that are essential for cell motility [16] , [21] . As eotaxin-1 upregulated ORMDL3 expression, we examined whether increased ORMDL3 expression in eosinophils may alter the actin cytoskeleton based on phalloidin staining. ORMDL3 -GFP-transfected eosinophils exhibited striking changes in the F-actin cytoskeleton. Although control-GFP-transfected cells demonstrated a distinct pattern of phalloidin binding localized to the cell periphery/margin, ORMDL3 -GFP-transfected cells exhibited irregular phalloidin binding all over the cell ( Fig. 2e ). The important role of the cytoskeleton in promoting activation-dependent cell shape changes required for cell motility [22] , [23] together with the ability of ORMDL3 to alter the F-actin cytoskeleton when overexpressed, prompted us to investigate whether ORMDL3 has a role in regulating eosinophil trafficking. Overexpression of ORMDL3 in eosinophils resulted in significantly increased eosinophil rolling on recombinant murine (rm) VCAM-1 under conditions of flow compared with cells transfected with control-GFP ( Fig. 2f ). ORMDL3 regulates integrin expression and cell adhesion The role of ORMDL3 in eosinophil trafficking was further validated by knockdown studies using ORMDL3 -specific small interfering RNA (siRNA). Treatment of eosinophils with ORMDL3 -siRNA resulted in a marked reduction in ORMDL3 mRNA expression by RT–PCR and protein expression by western blot analysis as well as immunofluorescence staining ( Fig. 3a ) without significantly affecting cell viability or proliferation relative to cells treated with control-siRNA ( Supplementary Table S2 ). Interestingly, knockdown of ORMDL3 had no effect on eosinophil rolling ( Supplementary Fig. S3a ). This could be due to redundant eosinophil-expressed adhesion molecules such as galectin-3 that can promote eosinophil rolling on VCAM-1 (ref. 24 ). However, a significant reduction in adhesion of ORMDL3 -siRNA-treated eosinophils to rm VCAM-1 and rm ICAM-1 was noted compared with control-siRNA-treated cells ( Fig. 3b ). Confocal microscopy studies after phalloidin staining revealed that control-siRNA-treated eosinophils adherent to VCAM-1 and ICAM-1 exhibited cell spreading with distinct cell polarization (leading edge formation and development of uropodia and filopodia) ( Fig. 3c , middle panel) similar to untreated cells ( Fig. 3c , left panel), whereas knockdown of ORMDL3 resulted in not only a reduced number of adherent cells but also limited cell spreading/polarization ( Fig. 3c , right panel). Quantitation of these changes in cell morphology revealed that a significantly larger percentage of ORMDL3 -siRNA-treated eosinophils adhered to VCAM-1 and ICAM-1 do not spread (retain a compact round cell body without leading edges) compared with control-siRNA-treated or untreated eosinophils ( Fig. 3d ) correlating with the number of adherent cells in adhesion assays ( Fig. 3b ). 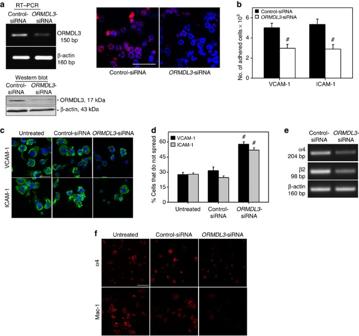Figure 3:ORMDL3-mediated eosinophil adhesion and regulation of integrin receptors α4 and β2. (a) Expression of ORMDL3 in BM-derived eosinophils transfected with control-siRNA orORMDL3-siRNA by RT–PCR (top left) as well as western blot (bottom) and immunofluorescence staining (top right) with antibodies against ORMDL3. Scale bar, 50 μm. (b) Adhesion of eosinophils treated with control-siRNA orORMDL3-siRNA to rm VCAM-1 and rm ICAM-1 under static conditions. (c) Changes in morphology ofORMDL3-siRNA-transfected eosinophils adherent on VCAM-1- or ICAM-1-coated cover-slips evaluated by confocal microscopy after phalloidin staining (right panels). Adherent control-siRNA-treated (middle panels) and untreated (media alone) eosinophils (left panels) are shown as controls. Scale bar, 20 μm. (d) Quantitation of changes in morphology of adherent eosinophils treated with control-siRNA,ORMDL3-siRNA or left untreated as in (c). The number of adherent cells in each field was counted and the number of cells in the field that do not spread and/or polarize (retain a round compact cell body without leading edges) were identified and expressed as a percentage of the total number of adhered cells. Five fields were counted for each cover-slip. (e) Expression of α4 and β2 integrins in eosinophils treated with control-siRNA orORMDL3-siRNA by RT–PCR. Expression of β-actin is shown as the internal control. (f) Expression of integrin α4 and Mac-1 (αM) by untreated (left panels), control-siRNA-treated (middle panels) andORMDL3-siRNA-treated (right panels) eosinophils adherent on VCAM-1 and ICAM-1, respectively, by immunofluorescence staining and confocal microscopy. Scale bar, 50 μm. Data shown in (a), (c), (e) and (f) are representative of two to three independent experiments with eosinophils from different mice. Combined data (mean±s.e.m.) of three experiments in triplicate in (b) and two experiments in duplicate in (d) are shown.#P<0.01 in (b) and (d) compared with control-siRNA. Statistical significance was determined by unpaired two-tailed Student’st-test. Figure 3: ORMDL3-mediated eosinophil adhesion and regulation of integrin receptors α4 and β2 . ( a ) Expression of ORMDL3 in BM-derived eosinophils transfected with control-siRNA or ORMDL3 -siRNA by RT–PCR (top left) as well as western blot (bottom) and immunofluorescence staining (top right) with antibodies against ORMDL3. Scale bar, 50 μm. ( b ) Adhesion of eosinophils treated with control-siRNA or ORMDL3 -siRNA to rm VCAM-1 and rm ICAM-1 under static conditions. ( c ) Changes in morphology of ORMDL3 -siRNA-transfected eosinophils adherent on VCAM-1- or ICAM-1-coated cover-slips evaluated by confocal microscopy after phalloidin staining (right panels). Adherent control-siRNA-treated (middle panels) and untreated (media alone) eosinophils (left panels) are shown as controls. Scale bar, 20 μm. ( d ) Quantitation of changes in morphology of adherent eosinophils treated with control-siRNA, ORMDL3 -siRNA or left untreated as in ( c ). The number of adherent cells in each field was counted and the number of cells in the field that do not spread and/or polarize (retain a round compact cell body without leading edges) were identified and expressed as a percentage of the total number of adhered cells. Five fields were counted for each cover-slip. ( e ) Expression of α4 and β2 integrins in eosinophils treated with control-siRNA or ORMDL3 -siRNA by RT–PCR. Expression of β-actin is shown as the internal control. ( f ) Expression of integrin α4 and Mac-1 (αM) by untreated (left panels), control-siRNA-treated (middle panels) and ORMDL3 -siRNA-treated (right panels) eosinophils adherent on VCAM-1 and ICAM-1, respectively, by immunofluorescence staining and confocal microscopy. Scale bar, 50 μm. Data shown in ( a ), ( c ), ( e ) and ( f ) are representative of two to three independent experiments with eosinophils from different mice. Combined data (mean±s.e.m.) of three experiments in triplicate in ( b ) and two experiments in duplicate in ( d ) are shown. # P <0.01 in ( b ) and ( d ) compared with control-siRNA. Statistical significance was determined by unpaired two-tailed Student’s t -test. Full size image As knockdown of ORMDL3 in eosinophils resulted in reduced cell adhesion and inhibition of activation-dependent (that is, adherent on VCAM-1 and ICAM-1) directed cell shape changes, we examined whether ORMDL3 regulates expression of adhesion molecules that are known to mediate eosinophil trafficking (rolling and adhesion). Knockdown of ORMDL3 in eosinophils resulted in decreased mRNA levels of α4 and β2, counter receptors for VCAM-1 and ICAM-1, respectively ( Fig. 3e ). Consistent with decreased mRNA levels of α4 and β2, immunostaining of ORMDL3 -silenced eosinophils adherent on VCAM-1 and ICAM-1 demonstrated decreased surface expression of α4 and Mac-1 (αM), respectively ( Fig. 3f , right panels), relative to untreated ( Fig. 3f , left panels) and control-siRNA-treated ( Fig. 3f , middle panels) eosinophils. Conversely, eosinophils overexpressing ORMDL3 demonstrated increased expression of α4 and β2 by RT–PCR ( Supplementary Fig. S3b ). mRNA levels of αM and αL as well as that of β1 remained unaffected in ORMDL3 -silenced eosinophils ( Supplementary Fig. S3c ), suggesting that the reduced surface expression of Mac-1 is most likely due to decreased expression of the β2 subunit by these cells. ORMDL3 regulates migration and CD48-mediated degranulation Cellular events such as adhesion and migration are known to be regulated by [Ca 2+ ] i levels through integrin activation and cytoskeletal changes [25] , [26] . Previous studies have demonstrated a role for ORMDL3 in regulating ER-mediated Ca 2+ homeostasis [10] , [27] . As our data suggest that ORMDL3 is involved in regulating cytoskeletal changes and adhesion of eosinophils, we examined whether [Ca 2+ ] i has a role in mediating these effects of ORMDL3 . Basal- and agonist (eotaxin-1)-induced [Ca 2+ ] i levels in control-siRNA-treated cells were significantly higher than in ORMDL3 -silenced eosinophils ( Fig. 4a ), and similar to levels in untreated cells ( Supplementary Fig. S4a ). This is in contrast to previous studies where knockdown of ORMDL3 in HEK293 and Jurkat T cells had no significant effect on basal cytosolic Ca 2+ levels [10] , [27] . This difference in the effect of ORMDL3 knockdown on basal [Ca 2+ ] i between our study and the previous studies may be due to the different cell types investigated (primary cells (eosinophils) versus transformed epithelial and T cell lines). Along with decreased agonist (eotaxin-1)-induced [Ca 2+ ] i levels, knockdown of ORMDL3 in eosinophils also significantly inhibited eotaxin-1-induced migration compared with eosinophils treated with control-siRNA or untreated eosinophils in in vitro chemotaxis assays ( Fig. 4b ). Conversely, eosinophils overexpressing ORMDL3 demonstrated increased migration towards eotaxin-1 compared with cells transfected with control-GFP, although statistical significance was not achieved ( Supplementary Fig. S4b ). The ability of ORMDL3 to regulate eosinophil migration was further validated in vivo where, in comparison with infused carboxyfluorescein succinimidyl ester (CFSE)-labelled control-siRNA-treated eosinophils, a reduced number (three-fold reduction) of CFSE-labelled ORMDL3 -siRNA-treated eosinophils were found to recruit to the inflamed peritoneum of mice exposed to thioglycollate ( Fig. 4c,d ). 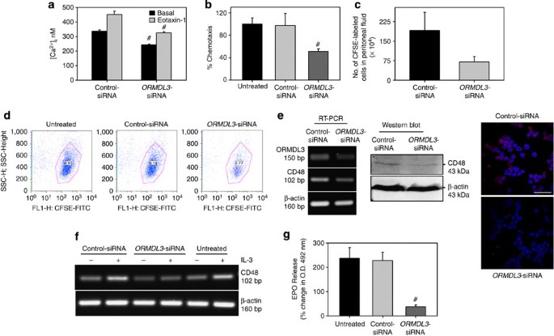Figure 4:ORMDL3-dependent eosinophil migration and CD48-mediated degranulation. (a) Basal and eotaxin-1 (100 nM)-induced [Ca2+]ilevels in eosinophils treated with control-siRNA (a total of 598 cells) orORMDL3-siRNA (a total of 870 cells) by digital video fluorescence imaging after loading with Fura-2 AM. (b) Chemotaxis of untreated, control-siRNA-treated andORMDL3-siRNA-treated eosinophils in response to eotaxin-1 (100 nM)in vitro. (c) Recruitment of infused CFSE-labelled control-siRNA- orORMDL3-siRNA-treated eosinophils to the peritoneum in a mouse model of thioglycollate (TG)-induced inflammation by flow cytometry. (d) Dot plots from a representative experiment showing recruitment of CFSE-labelled untreated, control-siRNA-treated andORMDL3-siRNA-treated eosinophils to the peritoneum of a TG-exposed mouse. The experiment was repeated three times with similar results (n=3 mice per condition). (e) Expression of CD48 in eosinophils treated with control-siRNA orORMDL3-siRNA by RT–PCR (left), western blot analysis (middle) and immunofluorescence staining (right). Scale bar, 50 μm. (f) CD48 expression after IL-3 treatment in control-siRNA-treated,ORMDL3-siRNA-treated and untreated eosinophils by RT–PCR. Expression of β-actin is shown as the internal control in panels (e,f). (g) EPO release by untreated, control-siRNA-treated andORMDL3-siRNA-treated eosinophils after activation with anti-CD48 by colorimetric assay expressed as per cent change in absorbance relative to treatment with control IgG. In the panels (a,b,g), combined data (mean±s.e.m.) of three experiments in duplicate or triplicate and in (c), combined data (mean±s.d.) of two experiments are shown. Data shown in (e) and (f) are representative of two to three independent experiments with eosinophils from different mice.#P<0.01 in the panels (a,g) and <0.05 in (b) compared with control-siRNA. Statistical significance was determined by unpaired two-tailed Student’st-test. Figure 4: ORMDL3-dependent eosinophil migration and CD48-mediated degranulation . ( a ) Basal and eotaxin-1 (100 nM)-induced [Ca 2+ ] i levels in eosinophils treated with control-siRNA (a total of 598 cells) or ORMDL3 -siRNA (a total of 870 cells) by digital video fluorescence imaging after loading with Fura-2 AM. ( b ) Chemotaxis of untreated, control-siRNA-treated and ORMDL3 -siRNA-treated eosinophils in response to eotaxin-1 (100 nM) in vitro . ( c ) Recruitment of infused CFSE-labelled control-siRNA- or ORMDL3 -siRNA-treated eosinophils to the peritoneum in a mouse model of thioglycollate (TG)-induced inflammation by flow cytometry. ( d ) Dot plots from a representative experiment showing recruitment of CFSE-labelled untreated, control-siRNA-treated and ORMDL3 -siRNA-treated eosinophils to the peritoneum of a TG-exposed mouse. The experiment was repeated three times with similar results ( n =3 mice per condition). ( e ) Expression of CD48 in eosinophils treated with control-siRNA or ORMDL3 -siRNA by RT–PCR (left), western blot analysis (middle) and immunofluorescence staining (right). Scale bar, 50 μm. ( f ) CD48 expression after IL-3 treatment in control-siRNA-treated, ORMDL3- siRNA-treated and untreated eosinophils by RT–PCR. Expression of β-actin is shown as the internal control in panels ( e , f ). ( g ) EPO release by untreated, control-siRNA-treated and ORMDL3 -siRNA-treated eosinophils after activation with anti-CD48 by colorimetric assay expressed as per cent change in absorbance relative to treatment with control IgG. In the panels ( a , b , g ), combined data (mean±s.e.m.) of three experiments in duplicate or triplicate and in ( c ), combined data (mean±s.d.) of two experiments are shown. Data shown in ( e ) and ( f ) are representative of two to three independent experiments with eosinophils from different mice. # P <0.01 in the panels ( a , g ) and <0.05 in ( b ) compared with control-siRNA. Statistical significance was determined by unpaired two-tailed Student’s t -test. Full size image Our observation that IL-3 induces ORMDL3 expression by eosinophils together with previous studies demonstrating that IL-3 can induce expression of CD48, a GPI-anchored protein involved in cellular activation, costimulation and adhesion of eosinophils [28] , prompted us to investigate whether ORMDL3 regulates CD48 expression. Relative to unstimulated (no IL-3) murine eosinophils treated with control-siRNA, ORMDL3 -silenced cells exhibited reduced CD48 mRNA expression by RT–PCR ( Fig. 4e , left) as well as protein expression by western blot analysis ( Fig. 4e , centre) and immunofluorescence staining ( Fig. 4e , right). Although exposure to IL-3 induced CD48 expression in eosinophils ( Supplementary Fig. S4c ), there was a marked inhibition of IL-3-induced CD48 mRNA expression in ORMDL3 -silenced eosinophils compared with untreated and control-siRNA-treated cells ( Fig. 4f ). Given that CD48 crosslinking on human eosinophils results in activation-dependent cell degranulation [28] , we examined whether ORMDL3 regulates CD48-induced degranulation of murine eosinophils ( Fig. 4g ). Activation of control eosinophils (treated with media containing transfection reagent without any siRNA) with anti-CD48 mAbs induced cellular degranulation as measured by eosinophil peroxidase (EPO) release. Activation with anti-CD48 after ORMDL3 knockdown resulted in a five-fold reduction in degranulation compared with control-siRNA-treated eosinophils. These results indicate that ORMDL3 is not only required for IL-3-induced expression of CD48 but also for activation-dependent (CD48-mediated) degranulation of eosinophils. Considering Th2 cytokines and chemokines exert various immunomodulatory effects on eosinophils [14] , it is interesting that IL-3, but not IL-5, induces ORMDL3 gene expression. Although the receptor for IL-3 and IL-5 share a β-chain [29] , our results suggest that the selective IL-3-induced upregulation of ORMDL3 is potentially via a IL-3R α-chain-specific mechanism and independent of common β-chain-mediated signalling in eosinophils. Likewise, induction of ORMDL3 gene expression by eotaxin-1, but not RANTES, although both chemokines can bind to CCR3 (refs 30 , 31 ), is suggestive of selective signalling mechanisms that potentially regulate ORMDL3 expression in eosinophils. In human eosinophils, eotaxin-1 is known to induce rapid activation of ERK, which is necessary for eotaxin-induced cytoskeletal rearrangement, chemotaxis and degranulation [16] , [17] , [32] . Overexpression of ORMDL3 in murine eosinophils was associated with increased levels of phosphorylated ERK (1/2), but not p38, which suggests association of specific MAP kinase signalling pathways with ORMDL3. Further, increased ORMDL3 expression was found to result in distinct cytoskeletal changes. Rearrangement of the cytoskeleton in response to a stimulus enables changes in cell shape/morphology (spreading and polarization), which are essential for cell trafficking (rolling and adhesion) and migration [22] , [23] . Indeed, eosinophils overexpressing ORMDL3 demonstrate increased rolling on VCAM-1 and migration. [Ca 2+ ] i acts as a biologically important second messenger after stimulation with cytokines and chemokines. ORMDL3 -silenced eosinophils had reduced basal and agonist-induced [Ca 2+ ] i levels relative to control cells. This function of ORMDL3 in regulating [Ca 2+ ] i can impact various functional responses in eosinophils that are driven by changes in [Ca 2+ ] i such as cytoskeletal reorganization and cell shape change/morphology, as well as modulation of integrin receptors, cell adhesion, migration and degranulation [33] , which were all affected in the present study in ORMDL3 -silenced eosinophils. Specifically, ORMDL3 knockdown studies resulted in reduced surface expression of α4 and Mac-1 along with decreased adhesion to VCAM-1 and ICAM-1 in eosinophils. Conversely overexpression of ORMDL3 resulted in increased α4 and β2 mRNA expression. This could potentially be through NF-κB activation and translocation as previous studies have shown that α4 expression in monocytes-derived dendritic cells [34] and β2 expression in eosinophils [20] is dependent on NF-κB activation/nuclear translocation. Further, with cell surface expression of CCR3 (receptor for eotaxin-1) remaining unaffected after ORMDL3 knockdown ( Supplementary Fig. S4d ), decreased migration of these cells suggests that signalling via ORMDL3 might be essential for eotaxin-1-induced eosinophil migration and recruitment to sites of inflammation in vivo . Induction of CD48 in eosinophils by IL-3 is β chain-independent [28] similar to IL-3-induced upregulation of ORMDL3 described here. ORMDL3 appears to have a role in regulating CD48. Not only IL-3-induced expression of CD48 but also CD48-mediated eosinophil degranulation (EPO release) is inhibited in ORMDL3 -silenced eosinophils. We postulate that ORMDL3 regulates CD48 via NF-κB activation in eosinophils based on the following lines of evidence. First, CD48 is known to be a target gene for NF-κB [35] . Second, IL-3 has been shown to induce NF-κB activation in eosinophils [20] . Third, in our studies, we show that IL-3 induces ORMDL3 as well as CD48, with expression of the latter being dependent on ORMDL3 and finally, overexpression of ORMDL3 is associated with NF-κB activation. In summary, we demonstrate for the first time a functional role for ORMDL3 in regulating eosinophil trafficking, recruitment and degranulation, which can promote airway eosinophilia and inflammation in allergic asthma. Further, our studies suggest that blockade of ORMDL3 may serve as a potential means to ameliorate eosinophilic inflammation during allergic asthma and other eosinophilic disorders. Mouse model of allergic airway inflammation C57BL/6 mice (male, 6–8 weeks) were challenged with 50 μg of A. alternata extract (Greer Laboratories Inc.) in 50 μl of PBS or PBS alone (control) intranasally on days 0, 3 and 6 under anaesthesia [36] . Mice were killed 18–24 h after the last challenge and evaluated for development of inflammation based on cellular infiltration in BALF and lung tissue [37] . In addition, lung tissue was harvested from C57BL/6 mice exposed to chronic challenge with ovalbumin [37] or acute challenge with cockroach antigen [21] . All animal studies were performed following standards and procedures approved by the Institutional Animal Care and Use Committee at the University of Minnesota. Immunohistology Expression of ORMDL3 in paraffin-embedded lung tissue sections was evaluated using rabbit anti-ORMDL3 (0.5 μg ml −1 for Alternaria -challenged, 2.5 μg ml −1 for ovalbumin- and cockroach antigen-challenged) generated against a synthetic peptide corresponding to internal sequence amino acids 56–85 of human ORMDL3 that is known to cross-react with mouse ORMDL3 (Abcam). Rabbit IgG (R&D systems) was used as the negative control. VECTASTAIN ABC kit containing biotinylated anti-rabbit secondary antibodies and avidin–biotin–HRP complex followed by peroxidase AEC substrate kit (both from Vector Laboratories) was used for detection. Lung tissue eosinophils were evaluated by staining for eosinophil-specific MBP with rat mAbs against murine MBP (2 μg ml −1 , provided by Dr J. Lee, Mayo Clinics Arizona, Scottsdale, AZ) [37] . Slides were examined under a Nikon Microphot EPI-FL microscope and images were captured with an Olympus DP71 camera. Immunofluorescence staining and confocal microscopy BALF cells from Alternaria -exposed mice cytocentrifuged onto glass slides were fixed, permeabilized, blocked with normal goat serum and simultaneously incubated overnight with antibodies against ORMDL3 (Abcam, 2.5 μg ml −1 ) and MBP (2 μg ml −1 ) at 4 °C. Rabbit IgG (for ORMDL3) and rat IgG (for MBP) were used as controls. Rhodamine Red-X-conjugated goat anti-rabbit and FITC-conjugated goat anti-rat (both at 7.5 μg ml −1 , Jackson ImmunoResearch Laboratories, Inc.) were used as secondary antibodies. With BM-derived eosinophils, cells on glass slides were fixed and blocked as described above. For detection of ORMDL3 expression, permeabilized cells were used, whereas for CD48 expression, cells were not permeabilized. Cells were incubated with antibodies against ORMDL3 (1.25 μg ml −1 ), mAb against CD48 (Santa Cruz Biotechnology, Inc., 1.25 μg ml −1 ) or control IgG followed by Rhodamine Red-X-conjugated goat anti-rabbit IgG (3 μg ml −1 ) or Rhodamine Red-X-conjugated donkey anti-mouse IgG (1.25 μg ml −1 , Jackson ImmunoResearch Laboratories). Slides were washed, mounted in medium containing 4′,6-diamidino-2-phenylindole (DAPI) and visualized by confocal microscopy at ambient temperature. Murine eosinophils Murine eosinophils were cultured from BM of C57BL/6 mice [38] . Cells between 12–14 days of culture differentiated based on Hema 3 staining and verified for expression of both MBP (by confocal microscopy with rat mAb against murine MBP at 2.5 μg ml −1 ) and Siglec-F (by flow cytometry with PE-conjugated rat anti-mouse Siglec-F at 5 μg ml −1 ) were used in studies. See Supplementary Methods for detailed culture conditions. RT–PCR and quantitative real-time RT–PCR Primers specific for murine ORMDL3 (5′-CACACGGGTGATGAACAGTC-3′ and 3′-TTTGCCTTGGTCTGGAGTCT-5′) were designed using Primer3 (v. 0.4.0, available online at http://frodo.wi.mit.edu/primers3/ ). Expression of CD48, CD18 (β2), CD49d (α4), CD11a (αL), CD11b (αM), CD29 (β1) and β-actin were examined using previously published primer sequences ( Supplementary Table S1 ). All primers were synthesized by Integrated DNA Technologies. PCR products were analysed by agarose gel (1.2%) electrophoresis. qPCR was carried out in a iQ5 multicolour real-time PCR detection System (Bio-Rad) using the same primer pair for ORMDL3 described above under the following conditions: initial denaturation at 95 °C for 2 min followed by 44 cycles of 95 °C for 15 s and 64 °C for 1 min. The relative amount of mRNA for each sample was calculated based on its threshold cycle, Ct, suggested by the software (IQ5 Optical System software) in comparison with the Ct of the housekeeping gene β-actin [37] . Results were expresses as fold change (2 ΔΔCT ) in expression after subtraction of internal β-actin control. Western blot analysis Murine BM-derived eosinophil lysates were analysed using antibodies against (i) ORMDL3 (0.16 μg ml −1 ), (ii) CD48 (0.2 μg ml −1 ), (iii) ERK (1/2) (0.01 μg ml −1 ), (iv) phospho-ERK (1/2), (0.12 μg ml −1 ), (v) p38 (0.026 μg ml −1 ), (vi) phospho-p38 (0.3 μg ml −1 ) (antibodies for (iii)–(vi) were from Cell Signaling Technology) and (vii) β-actin (BD Transduction Laboratories, 0.06 or 0.12 μg ml −1 ). Lung tissue lysates from PBS and Alternaria -exposed mice prepared in RIPA buffer containing protease and phosphatase inhibitors were examined for ORMDL3 expression as described for BM eosinophils. Expression of β-actin was monitored as an internal control in all cases and detection was carried out using secondary antibodies appropriate for the detection system used. See Supplementary Methods for experimental details. Representative full-length western blots are shown in the Supplementary Information ( Supplementary Figs S5,S6 ). Expression of recombinant ORMDL3 Full-length cDNA encoding the human ORMDL3 gene (Thermo Scientific Open Biosystems) was cloned into pET-28a vector containing a His tag, while full-length cDNA encoding the mouse ORMDL3 gene (Thermo Scientific Open Biosystems) was cloned into pGEX-6p-2 vector containing a GST tag. The resulting expression plasmids of the human or mouse ORMDL3 gene were transformed into E. coli Rosetta (DE3) pLysS cells. IPTG (1 μM)-induced recombinant bacteria were lysed in RIPA buffer containing protease inhibitors and 1 mM DTT and expression of His-tagged or GST-tagged ORMDL3 in the bacterial lysates was analysed by western blot analysis using polyclonal antibodies against ORMDL3. Overexpression and knockdown of ORMDL3 Full-length cDNA for ORMDL3 was cloned into pEGFP-N1 using standard cloning procedures. BM-derived mouse eosinophils were transfected with pEGFP-N1 containing cDNA for ORMDL3 ( ORMDL3- GFP) or with the empty vector (control-GFP) using Trans IT-2020 DNA transfection reagent (Mirus Bio LLC) as recommended by the manufacturer. Transfected cells cytocentrifuged onto glass slides, fixed, mounted in DAPI were evaluated by confocal microscopy and by RT–PCR. BM-derived eosinophils were transected with siRNA specific for ORMDL3 ( ORMDL3 -siRNA) or scrambled siRNA (control-siRNA, both from Santa Cruz Biotechnology, Inc.) using INTERFERin siRNA transfection reagent (Polyplus-transfection) according to the manufacturer’s recommendations. Cells were assessed for knockdown of ORMDL3 expression by RT–PCR and western blot. Cell number and viability based on Trypan blue exclusion was assessed before and after transfection. ER localization of ORMDL3 Eosinophils were treated with ER-Tracker Red for live-cell ER labelling (Invitrogen, 1 μM) according to the manufacturer, fixed with 4% paraformaldehyde, cytocentrifuged onto glass slides and evaluated by confocal microscopy. Assessment of cytoskeleton Eosinophils were cytocentrifuged onto glass slides, air dried, permeabilized with 4% paraformaldehyde containing 0.5% saponin and 2.5 U ml −1 rhodamine-conjugated phalloidin (Invitrogen) [21] and evaluated by confocal microscopy. Induction of ORMDL3 and CD48 expression BM-derived eosinophils (1 × 10 6 per well) were suspended in culture medium alone or medium containing IL-5, IL-3 (both from PeproTech), RANTES-1 (R&D Systems, all at 100 ng ml −1 ) or eotaxin-1 (PeproTech, 100 nM) for 2 h at 37 °C and 5% CO 2 after which cells were analysed for ORMDL3 mRNA expression by RT–PCR and qPCR. To evaluate CD48 mRNA expression, eosinophils were treated with IL-3 as described above. For protein expression, eosinophils were treated with IL-3 for 12 h and then examined for ORMDL3 and CD48 by western blot analysis followed by densitometry using ImageJ (for ORMDL3). In vitro flow chamber assay Rolling of BM-derived eosinophils (1–2 × 10 5 per ml) on rm VCAM-1-coated cover-slips under conditions of flow (1 ml min −1 , wall shear stress ~1.0–2.0 dynes cm −2 ) was evaluated in an in vitro parallel plate flow chamber [38] . Interaction of the infused eosinophils with VCAM-1 was observed using a Leitz Wetzlar inverted microscope and images were recorded for subsequent offline analysis to manually determine the number of cells demonstrating multiple discrete interruptions and flow slowly (rolling) relative to non-interacting cells. Results were expressed as the number of rolling cells per min. Adhesion assay Adhesion of BM-derived eosinophils to rm VCAM-1 and rm ICAM-1 was evaluated using static adhesion assays [39] . Cells labelled with 1 μM Calcein-AM (Invitrogen) were added to 96-well plates coated with rm VCAM-1 (5 μg ml −1 ) or rm ICAM-1 (10 μg ml −1 ). After washing to remove non-adherent cells, the number of adherent cells was quantitated using a FLUOStar Optima microplate reader (BMG Labtech) at an excitation wavelength of 485 nm and an emission of 520 nm against a generated standard curve of labelled eosinophils. Cell morphology and adhesion molecule expression Eosinophils were allowed to adhere to rm VCAM-1- or ICAM-1-coated cover slips for 30 min. After washing with PBS to remove non-adherent cells, adhered cells were fixed with 4% paraformaldehyde, permeablized and stained with Alexa Fluor 488 Phalloidin (Invitrogen) and visualized by confocal microscopy [39] . To quantitate differences in cell morphology, the number of adherent cells in a given field of each cover-slip was counted and the number of cells in the field that do not spread (retain a compact round cell body without leading edges) were identified and expressed as a percentage of the total number of adhered cells. Five fields were counted for each cover-slip. α4 and Mac-1 (αM) expression by eosinophils adhered on rm VCAM-1 and rm ICAM-1, respectively, was evaluated by confocal microscopy after staining with antibodies against α4 (5 μg ml −1 , Santa Cruz Biotechnology, Inc.) and Mac-1 (10 μg ml −1 , eBiosciences, Inc.) [39] . NF-κB translocation Eosinophils cytocentrifuged onto glass slides were fixed, permeabilized, blocked and incubated overnight at 4 °C with polyclonal antibodies against phospho-NF-κB p65 (Santa Cruz Biotechnology, Inc., 1 μg ml −1 ) followed by Rhodamine Red-X-conjugated goat anti-rabbit IgG (Jackson ImmunoResearch Laboratories, Inc., 1:1,000) [40] , stained with DAPI and then examined by confocal microscopy. Measurement of intracellular calcium concentration Basal and agonist (eotaxin-1 (100 nM))-induced [Ca 2+ ] i levels in eosinophils was determined using the permeant Ca 2+ indicator dye Fura-2AM (Invitrogen) by real-time digital video fluorescence imaging [38] , [41] . See Supplementary Methods for experimental details. In vitro migration assay Migration of eosinophils in response to murine eotaxin-1 (100 nM) was evaluated in 96-well Transwell Chambers as described previously [39] . Media alone served as the control to record background migration. The number of migrated cells per well was expressed as per cent migration relative to control (untreated) eosinophils after subtraction of background migration. In vivo migration of eosinophils Eosinophils were labelled with carboxyfluorescein succinimidyl ester (CSFE, Invitrogen) and infused (10 × 10 6 cells) into wild-type mice 13 h after peritoneal inflammation had been induced by injecting thioglycollate as described [38] . Two hours after cell infusion, the peritoneal cavity was lavaged and the number of cells recovered was counted. Peritoneal cells were analysed by flow cytometry to determine the number of CFSE-positive cells (that is, infused eosinophils). Cell activation and EPO release assay Eosinophils (2 × 10 5 per 200 μl) were incubated with anti-mouse CD48 mAb (BioLegend) or control hamster IgG (BioLegend) at 37 °C for 2 h in culture media containing transfection reagent without any siRNA after which EPO in supernatants was determined by colorimetric assay. Results are expressed as per cent change in absorbance relative to treatment with control IgG after subtraction of background. Statistical analysis Data are presented as mean±s.e.m. unless otherwise stated. Statistical significance between two groups was determined using a two-tail unpaired Student’s t -test. A P -value <0.05 was considered as significant. How to cite this article: Ha, S.G. et al. ORMDL3 promotes eosinophil trafficking and activation via regulation of integrins and CD48. Nat. Commun. 4:2479 doi: 10.1038/ncomms3479 (2013).